Polymorphism in a high-entropy alloy Polymorphism, which describes the occurrence of different lattice structures in a crystalline material, is a critical phenomenon in materials science and condensed matter physics. Recently, configuration disorder was compositionally engineered into single lattices, leading to the discovery of high-entropy alloys and high-entropy oxides. For these novel entropy-stabilized forms of crystalline matter with extremely high structural stability, is polymorphism still possible? Here by employing in situ high-pressure synchrotron radiation X-ray diffraction, we reveal a polymorphic transition from face-centred-cubic ( fcc ) structure to hexagonal-close-packing ( hcp ) structure in the prototype CoCrFeMnNi high-entropy alloy. The transition is irreversible, and our in situ high-temperature synchrotron radiation X-ray diffraction experiments at different pressures of the retained hcp high-entropy alloy reveal that the fcc phase is a stable polymorph at high temperatures, while the hcp structure is more thermodynamically favourable at lower temperatures. As pressure is increased, the critical temperature for the hcp -to- fcc transformation also rises. Polymorphism, which refers to the ability of a solid material to exist in more than one crystal structure, is widely observed in many materials including polymers [1] , minerals [2] , [3] , [4] and metals [5] , [6] , [7] , [8] . The polymorphic transition is a well-known yet critical phenomenon in nature and surprisingly, polymorphs with identical compositions can have different physical, chemical and mechanical properties due to different structural characteristics, which have attracted considerable attention over the last few decades [9] , [10] , [11] . Pressure and temperature are usually controlling parameters for inducing these transitions by altering the atomic and/or electronic structures and creating novel materials. For example, carbon can take on graphite and diamond under different pressures and temperatures. Recently, a new alloy design concept based on entropic contributions to the thermodynamic landscape, rather than cohesive energy, was proposed [12] , [13] , which was subsequently extended to non-metallic systems such as multicomponent oxides [14] . This strategy was explored by deliberately incorporating five or more elemental species into a single lattice with random site occupancy. Due to the engineered configuration disorder, these entropy-stabilized solid solution alloys, that is, high-entropy alloys (HEAs), usually show a single-phase structure with high symmetry and extremely attractive properties [15] , [16] , [17] , [18] , [19] , [20] , [21] . Among various reported HEAs in literature, the equiatomic CoCrFeMnNi alloy (also termed as Cantor’s alloy) [12] , [13] is a prototype fcc (face-centred-cubic) HEA, which possesses ultrahigh fracture toughness and large ductility, even at cryogenic temperatures [19] , [22] , [23] . It is generally believed that HEA lattices are severely distorted and atomic diffusion is extremely sluggish due to the chemical complexity and packing disorder [24] , [25] . Consequently, HEAs have exceptionally high microstructural stability [26] , [27] . Many studies also demonstrate that the CoCrFeMnNi HEA can maintain its fcc structure over a large temperature range from cryogenic temperatures up to the melting temperature without any polymorphic phase transition [19] , [22] , [28] . Considering the extensive polymorphism in the typical constituent elements of HEAs, such as Fe, Co and Mn [29] , an intriguing question is naturally raised: when metallic alloys are made in the entropy-stabilized form of crystalline matter with high structural stability, is polymorphism still possible? More recently, long-term annealing experiments at intermediate temperatures revealed that different crystalline phases could precipitate out of the CoCrFeMnNi HEA fcc matrix [27] , [30] , [31] . Moreover, finite-temperature ab initio simulation results suggest that the free energy of the hcp (hexagonal-close-packing) crystallographic lattice in the CoCrFeMnNi HEA may be lowest at room temperature, compared with that of its bcc (body-centerd-cubic) and fcc counterparts [32] , [33] . All these results cast doubt on the high structural stability of HEA lattices, which is obviously a critical and vital problem for our understanding and applications of these newly developed metallic materials and multicomponent oxides. However, until now the predicted hcp phase of the CoCrFeMnNi HEA has not been observed in any experiments and the question of viable polymorphism remains unanswered. In this work, we employed an in situ high-pressure synchrotron radiation X-ray diffraction (XRD) technique and discovered a polymorphic transition from fcc to hcp in the prototype CoCrFeMnNi HEA under hydrostatic compression at room temperature. The phase transition is sluggish, it starts at ∼ 22 GPa and almost completes at ∼ 41 GPa, and the hcp phase could be retained when the pressure was totally released, which is the first synthesis of the CoCrFeMnNi HEA with an hcp structure at ambient conditions. Our in situ laser/resistive heating XRD experiments at different pressures show an inverse transition from hcp back to fcc at elevated temperatures and reveal that the fcc phase is stable at high temperatures while the hcp structure is more thermodynamically favourable at relatively lower temperatures. Our findings indicate that this fcc HEA is a thermodynamically metastable polymorph obtained by kinetic constraints and the thermodynamically favourable hcp structure is relatively difficult to attain. Microstructure and compositional analysis The CoCrFeMnNi HEA sample was synthesized using a gas-atomization technique [34] . The gas-atomized powders are spherical particles with a typical size ranging from a few microns to tens of microns, which are appropriate for high-pressure experiments ( Supplementary Fig. 1 ). These particles are polycrystalline with a grain size ranging from submicron to a few microns (the inset of Supplementary Fig. 1 ). The chemical and energy dispersive X-ray spectroscopy analyses confirm that the composition of the as-atomized CoCrFeMnNi HEA is close to the nominal composition, and there are no compositional changes after the high-pressure XRD tests ( Supplementary Fig. 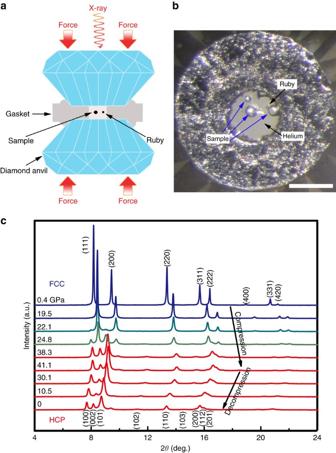Figure 1: Experimental set-up and thein situhigh-pressure XRD patterns of the CoCrFeMnNi HEA in a DAC during compression and decompression at room temperature. (a,b) A schematic illustration of the DAC used to generate high-pressure on tiny samples for thein situhigh-pressure experiment. (c) XRD patterns as a function of pressure obtained during compression and decompression with a X-ray wavelengthλ=0.2952 Å. The initial phase is indexed to anfcclattice, whereas the new phase synthesized above 22 GPa is well indexed to anhcplattice. Intensity mismatch of the standardfccandhcpstructures is caused by the relatively large grains in the samples. The scale bar inbrepresents 100 μm. 2 and Supplementary Table 1 ). In situ high-pressure synchrotron XRD at room temperature Hydrostatic pressure up to ∼ 41 GPa was applied to the tiny CoCrFeMnNi HEA particles using a diamond anvil cell (DAC). The experimental set-up of the DAC and the sample loading image are shown in Fig. 1a,b , respectively. More details can be found in Methods. The structural evolution of the CoCrFeMnNi HEA during compression was monitored by high-brightness synchrotron radiation XRD through two transparent diamond anvils of the DAC. The XRD patterns collected from both the compression and decompression processes are shown in Fig. 1c . The initial HEA sample has an fcc single-phase structure, which remains stable up to 19.5 GPa. All diffraction reflections shift towards higher 2 θ values, which is an expected result of the pressure-induced volume decrease. Once the pressure approaches 22.1 GPa, extra diffraction peaks beside the (111) peak of fcc appeared (indicated by red triangles in Fig. 1c ), suggesting the occurrence of a phase transition. With further increasing pressure, the intensity of the fcc peaks was obviously lowered, while that of the new diffraction peaks increased appreciably. The transition was sluggish, the fcc and new phase coexisted over large pressure range. At the maximum pressure of ∼ 41 GPa, the diffraction reflections mainly corresponded to the new phase while only minute residual fcc phase remained. During decompression, surprisingly the phase transition was irreversible. The newly formed phase was completely retained down to ambient pressure. All the new phase peaks were well indexed as crystallographic reflections of an hcp lattice (space group P6 3 /mmc ), which revealed an fcc -to- hcp transition under high-pressure in the prototype CoCrFeMnNi HEA ( Table 1 and Supplementary Fig. 3 ). Detailed information about their structure, such as the interplanar d -spacing ( Fig. 2a ) and unit cell volume ( Fig. 2b ) as a function of the applied pressure, was obtained by fitting the measured compression and decompression XRD patterns using the Le Bail method in the standard GSAS package [35] . The c / a ratio of the hcp phase remained almost constant at 1.62±0.01 during both compression and decompression. These two sets of volume data in Fig. 2b can be well fitted by a third-order Birch-Murnaghan isothermal equation of state (EOS) [36] , with the isothermal bulk modulus B 0 =153.9±3.0 GPa and its pressure derivative =4.9±0.7 for the fcc phase and B 0 =150.2±4.6 GPa and =6.2±0.5 for the hcp phase. The bulk moduli obtained in this work are consistent with previous experimental results [28] on the fcc phase and simulation results [33] , [37] on both the fcc and hcp phases. The two phases exhibit no obvious difference in both volume and bulk modulus. It should be noted that the grain size of the sample is still not small enough to obtain smooth diffraction rings, as compared with the tiny X-ray beam size (2.5 × 4 μm 2 ). Therefore, the relative intensity of the different peaks is not statistically reliable for the Rietveld refinement to accurately derive the volume fractions of the fcc and hcp phases during the transition. Alternatively, by assuming the phase fraction is proportional to the area of corresponding diffraction peaks, such as the fcc -(200) and hcp -(101) peak areas in Fig. 1c , the volume fraction of hcp as a function of pressure during both compression and decompression can be roughly estimated ( Supplementary Fig. 4 ). The results in Supplementary Fig. 4 confirm that the transition is sluggish over a wide pressure range and irreversible with an almost constant volume fraction of hcp during the decompression. Figure 1: Experimental set-up and the in situ high-pressure XRD patterns of the CoCrFeMnNi HEA in a DAC during compression and decompression at room temperature. ( a , b ) A schematic illustration of the DAC used to generate high-pressure on tiny samples for the in situ high-pressure experiment. ( c ) XRD patterns as a function of pressure obtained during compression and decompression with a X-ray wavelength λ =0.2952 Å. The initial phase is indexed to an fcc lattice, whereas the new phase synthesized above 22 GPa is well indexed to an hcp lattice. Intensity mismatch of the standard fcc and hcp structures is caused by the relatively large grains in the samples. The scale bar in b represents 100 μm. Full size image Table 1 Unit-cell parameters and d -spacings of the different ( hkl ) planes of both the fcc and hcp CoCrFeMnNi HEAs at different pressures. 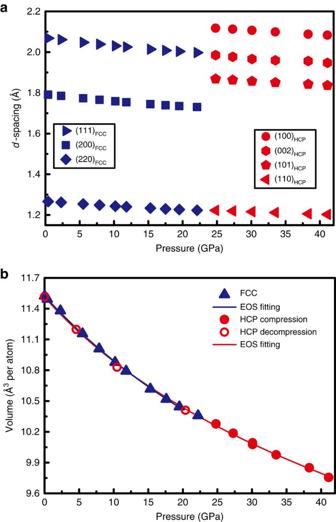Figure 2: Pressure dependence of the CoCrFeMnNi HEAd-spacings and volume. (a) The pressure dependence of thed-spacings associated with the major Bragg peaks offcc(shown in blue symbols) andhcp(shown in red symbols), respectively. The error bars are smaller than the symbol sizes. (b) The average volume per atom for both thefcc(blue triangles) andhcpphases (red solid circles for compression and red open circles for decompression) are calculated as a function of pressure. The volume data can be well fitted using the third-order Birch-Murnaghan EOS for bothfcc(blue solid line) andhcp(red solid line). The EOS offccandhcpalmost coincides with each other, showing no obvious volume difference at any given pressure. Full size table Figure 2: Pressure dependence of the CoCrFeMnNi HEA d -spacings and volume. ( a ) The pressure dependence of the d -spacings associated with the major Bragg peaks of fcc (shown in blue symbols) and hcp (shown in red symbols), respectively. The error bars are smaller than the symbol sizes. ( b ) The average volume per atom for both the fcc (blue triangles) and hcp phases (red solid circles for compression and red open circles for decompression) are calculated as a function of pressure. The volume data can be well fitted using the third-order Birch-Murnaghan EOS for both fcc (blue solid line) and hcp (red solid line). The EOS of fcc and hcp almost coincides with each other, showing no obvious volume difference at any given pressure. Full size image In situ laser/resistive heating synchrotron radiation XRD The irreversibility of the phase transition questions the relative stability of the fcc and hcp phases. To clarify this, in situ heating XRD studies were carried out at different pressures on the synthesized hcp phase. At ambient pressure, the hcp sample was sealed in a resistive heating DAC using silicone oil to prevent oxidation of the tiny sample. The hcp phase remained stable up to 633 K at ambient pressure, and almost completely transformed back to fcc when heated up to 723 K ( Supplementary Fig. 5 ). Once the pressure was increased, the critical transition temperature significantly increased, which is beyond the limit of the resistive heating DAC. Therefore, a double-sided Nd:YLF laser heating system coupled with a DAC was employed to heat the hcp phase at higher pressures of 6, 14 and 26 GPa. As an example, Fig. 3a presents the in situ laser heating XRD patterns collected at 26 GPa. With continuous heating above ∼ 1,400 K at 26 GPa, the fcc phase started to gradually grow at the expense of the hcp phase. Therefore, the temperature of ∼ 1,400 K was determined to be the critical temperature ( fcc -in) for the phase transition. Based on four critical transition temperatures determined at different pressures, a boundary is proposed in Fig. 3b . 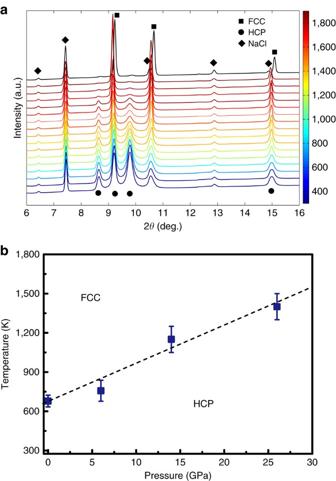Figure 3:In situlaser heating XRD of the CoCrFeMnNi HEA at different pressures. (a) The XRD patterns as a function of temperature from room temperature to 1,850 K with an X-ray wavelength of∼0.3220 Å. The intensity of the majorhcppeaks is almost constant below 1,400 K, but starts to gradually decrease during continuous heating above∼1,400 K, indicating the critical transition temperature occurs at∼1,400 K. (b) The temperature and pressure metastability boundary (not the equilibrium phase boundary) of thehcpCoCrFeMnNi HEA. The critical transition temperature is determined as the first appearance temperature of thefccphase from thehcpphase (synthesis curve of thefccphase) during heating at different pressures and it increases with pressure. The error bars of temperatures were estimated by the fitting errors of the blackbody radiation spectra and the temperature difference between two sides of the sample. Figure 3: In situ laser heating XRD of the CoCrFeMnNi HEA at different pressures. ( a ) The XRD patterns as a function of temperature from room temperature to 1,850 K with an X-ray wavelength of ∼ 0.3220 Å. The intensity of the major hcp peaks is almost constant below 1,400 K, but starts to gradually decrease during continuous heating above ∼ 1,400 K, indicating the critical transition temperature occurs at ∼ 1,400 K. ( b ) The temperature and pressure metastability boundary (not the equilibrium phase boundary) of the hcp CoCrFeMnNi HEA. The critical transition temperature is determined as the first appearance temperature of the fcc phase from the hcp phase (synthesis curve of the fcc phase) during heating at different pressures and it increases with pressure. The error bars of temperatures were estimated by the fitting errors of the blackbody radiation spectra and the temperature difference between two sides of the sample. Full size image The structural stability of the prototype CoCrFeMnNi HEA has been extensively studied in a wide temperature range from 55 K to its melting temperature of ∼ 1,600 K at ambient pressure [19] , [31] , [37] , [38] but to our knowledge, no polymorphic transition has been observed. Conversely, high-pressure studies remain a virgin area in HEAs. In this work, using in situ high-pressure XRD techniques, we observed the first polymorphic transition from fcc to hcp in the CoCrFeMnNi HEA, as shown in Fig. 1c . Therefore, some critical questions are how and why can an hcp HEA form at high-pressure and can it be maintained at ambient conditions? According to the d -spacing of the main reflections of both fcc and hcp (that is, (111) and (220) of fcc , and (100), (002), (101) and (110) of hcp , as a function of pressure shown in Fig. 2a ), it is clear that the hcp -(002) and hcp -(110) planes inherit the fcc -(111) and fcc -(220) planes, respectively. In addition, Fig. 2b shows no obvious volume collapse during the transition; both the fcc and hcp phases seem to have almost the same volume per atom and bulk modulus. This is similar to many other fcc to hcp martensitic transitions, such as in cobalt [39] or xenon [40] , which also show weak first-order features. It is well known that the fcc and hcp lattices only differ in the stacking sequence of the close packing layers, for example, the fcc and hcp crystal lattices follows the pattern of ABCABCABC…along the fcc [111] direction and ABABAB…along the hcp [001] direction, respectively. The hcp structure can be readily obtained locally from a fcc structure by introducing stacking faults. And it can be easily realized in the current HEA because recent experiment [41] and simulations [37] , [41] have confirmed that it indeed has a low staking fault energy of ∼ 20 mJ m −2 . However, the detailed mechanism of this transition could be much complex since the stacking faults, dislocations, and twining events may be all involved, and the magnetic states and volume (high pressure tuning) of the HEA alloy could also affect the transition behaviour [32] , [33] , [42] , [43] . As shown in Fig. 3 , the results of the in situ heating XRD experiments at different pressures explicitly demonstrate that the hcp phase of the CoCrFeMnNi HEA is relatively stable at low temperatures and high pressures, while the fcc phase is actually stable at higher temperatures and lower pressures, showing a boundary in between them with a positive slope. Using ab initio calculations, Ma et al . [32] actually revealed that thermodynamically, the CoCrFeMnNi HEA prefers the hcp structure below 340 K at ambient pressure and paramagnetic state while the fcc phase dominates at higher temperatures, which is qualitatively consistent with our experimental observations. It should be noted that in our experiment the phase transitions were sluggish and irreversible, suggesting high energy barriers between the hcp and the fcc phases, therefore overshooting often exists. It is difficult to determine the real equilibrium phase boundary (that is, the Clapeyron coexistence curve) experimentally. The curve in Fig. 3b is actually a synthesis curve showing the first appearance of the fcc phase ( fcc -in) from the hcp phase. During cooling, the fcc phase was fully recovered to room temperature showing a large metastability range. The real equilibrium phase boundary between fcc and hcp may be much lower than 633 K observed in experiments. According to Ostwald’s Rule [44] , high-temperature polymorphs often form first during cooling/crystallization. In other words, with conventional preparation techniques such as melt casting and atomization, the CoCrFeMnNi HEA always forms the fcc structure first, and when cooled down to room temperature, the transition from fcc to hcp likely depends on the entire complex γ -surface and could be kinetically hindered [32] , [42] , [45] . However, nano-twinning has been observed in the CoCrFeMnNi HEA at cryogenic temperatures (77 K) (ref. 19 ). This observation indicates that the stacking fault energy may diminish with decreasing temperature, which could facilitate the sliding needed for a displacive phase transition from fcc to hcp [32] . Recent theoretical work studied the stacking fault energy as a function of temperature in the CoCrFeMnNi HEA and confirmed this speculation [33] , [37] . Compared with temperature, pressure is a more powerful parameter in terms of decreasing the volume, tuning packing and energy state of a sample. The polymorphic transition from fcc to hcp unveiled in this work demonstrates that high-pressure can help overcome the kinetic barrier between hcp and fcc HEAs. Since the hcp CoCrFeMnNi HEA is more thermodynamically stable than the fcc polymorph at lower temperatures, the hcp phase can be retained after pressure release, and this hcp phase may have excellent mechanical properties at cryogenic temperatures. The polymorphic transition discovered in this work is by no means limited to this specific CoCrFeMnNi HEA, and we expect that this behaviour could be general in various HEAs at certain pressure and temperature conditions. Therefore, our results contribute to understanding of thermodynamics and kinetics in HEA systems. Moreover, the relative stability of the fcc and hcp phases of hard spheres is a long-standing problem in statistical physics. Since the fcc and hcp have identical packing densities and close free energy, the transition between fcc and hcp is believed to be entropy dominated. Therefore, the fcc - hcp transition in HEAs with extremely high entropy could provide ideal model systems for understanding fundamental questions about fcc and hcp packing [46] . Furthermore, we noticed that both the fcc and hcp can coexist over a wide pressure range ( ∼ 22 to ∼ 41 GPa), which could be attributed to the very similar free energy of the fcc and hcp phases and/or the large energy barrier between them. Decompression from different maximum pressures between ∼ 22 and ∼ 41 GPa in our repeated experiments successfully obtains fcc / hcp composites with tunable fractions after pressure release. As recently reported, the fcc-hcp dual-phase Fe 50 Mn 30 Co 10 Cr 10 composites, which undergo a strain-induced martensitic transformation of the initial fcc phase, exhibits outstanding mechanical properties that are much better than its monolithic counterpart [15] . However, no such dual phase composite has ever been observed in an equiatomic multicomponent HEA system with maximization entropy. According to the stability curve established in this work, the transition pressure could be largely decreased at cryogenic temperatures. Therefore, our results suggest new avenues for tailoring HEAs properties in their near infinite compositional space for novel applications via polymorphic transition-induced HEA composites. Sample preparation The polycrystalline CoCrFeMnNi HEA in our work was synthesized by a previously reported gas-atomization method [34] . Alloy ingots with a nominal composition of Co 20 Cr 20 Fe 20 Mn 20 Ni 20 were melted in an induction-heated vacuum furnace. The melt was then injected through a ceramic tube into the atomization chamber filled with high purity Ar gas. The atomization pressure was set at 4 MPa. The melt droplets cooled down and solidified into powder. The powder was then collected and sieved. Microstructure and chemistry characterization The composition of the gas-atomized powder was analysed with a titration method, and the oxygen content of the powder was determined by a fusion method on a Leco O/N analyser. The microstructure of the as-atomized specimens was characterized using a Zeiss Supra 55 scanning electron microscope operated at 15 kV with an energy dispersive spectrometer. In situ high-pressure synchrotron XRD at room temperature In situ high-pressure angle-dispersive XRD experiments were mainly performed at the beamline 13-ID-D, Advanced photon source (APS), Argonne National Laboratory (ANL). A monochromatic X-ray beam with a wavelength of 0.2952 Å was focused by a Kirkpatrick-Baez (KB) mirror system down to approximately 2.5 × 4 μm 2 , in a rectangular shape at the rotation centre of the sample stage. The detector position and orientation were calibrated using the LaB 6 standard. High-pressure was generated using a symmetric DAC with a 400 μm diameter culet. The gasket was T301 stainless steel that was pre-indented down to a thickness of ∼ 42 μm. A 180 μm hole was drilled as the sample chamber by a laser drilling system at the centre of the gasket indention. A few polycrystalline CoCrFeMnNi balls with a diameter of approximately 20 μm were selected and loaded into the DAC, along with a tiny ruby ball beside the samples to calibrate pressure. Helium was loaded into the DAC at sector 13, APS, ANL, as the hydrostatic pressure-transmitting medium. Figure 1b shows the image of the sample with helium loaded at 0.4 GPa. The pressure fluctuation estimated before and after each exposure was found to be less than 0.2 GPa. The background scattering was collected at each pressure by shining the X-ray beam on the empty area inside the sample chamber, which only passed through helium and two diamond anvils. Two-dimensional (2D) diffraction images were collected with a Mar165 charge-coupled device detector (pixel size: 79 × 79 μm 2 ) and the exposure time was set at 2 s. One-dimensional (1D) XRD patterns were obtained by integrating the 2D images along the azimuth angle from 0° to 360° with Dioptas software [47] . The resulting diffraction patterns were refined via Le Bail refinement using the GSAS package [35] . In situ resistive/laser heating XRD at different pressures To check the structural stability of the CoCrFeMnNi HEA hcp phase, in situ heating XRD experiments were conducted. Resistive heating up to 723 K in a DAC was performed on the high-pressure recovered hcp HEA sample at the beamline 12.2.2 of the Advanced Light Source, Lawrence Berkeley National Laboratory. The hcp -structured CoCrFeMnNi HEA for the heating experiment was synthesized by compressing the original fcc -structured CoCrFeMnNi HEA to 35 GPa and then decompressing it to ambient pressure in a DAC at room temperature. The wavelength of the X-ray was ∼ 0.4959 Å, and the beam size was 20 × 20 μm 2 . 2D XRD images were collected using a Mar345 image plate. To achieve higher temperatures and study the stability the hcp phase at higher pressures, a complementary online laser heating system coupled with DACs at the beamline 13-ID-D, APS, ANL was employed to perform double-sided laser heating on the hcp phased sample [48] . The wavelength of the X-ray was ∼ 0.3220 Å. NaCl was used as the pressure-transmitting medium, pressure standard and thermal insulator layers. Three pressure points of 6, 14 and 26 GPa were tested. Temperatures were determined by fitting the blackbody radiation spectra of the heated sample on both sides to the Planck radiation function. Data availability The data that support the findings of this study are available from the corresponding authors upon request. How to cite this article: Zhang, F. et al . Polymorphism in a high-entropy alloy. Nat. Commun. 8 , 15687 doi: 10.1038/ncomms15687 (2017). Publisher’s note : Springer Nature remains neutral with regard to jurisdictional claims in published maps and institutional affiliations.